Structural basis for potentiation by alcohols and anaesthetics in a ligand-gated ion channel Ethanol alters nerve signalling by interacting with proteins in the central nervous system, particularly pentameric ligand-gated ion channels. A recent series of mutagenesis experiments on Gloeobacter violaceus ligand-gated ion channel, a prokaryotic member of this family, identified a single-site variant that is potentiated by pharmacologically relevant concentrations of ethanol. Here we determine crystal structures of the ethanol-sensitized variant in the absence and presence of ethanol and related modulators, which bind in a transmembrane cavity between channel subunits and may stabilize the open form of the channel. Structural and mutagenesis studies defined overlapping mechanisms of potentiation by alcohols and anaesthetics via the inter-subunit cavity. Furthermore, homology modelling show this cavity to be conserved in human ethanol-sensitive glycine and GABA(A) receptors, and to involve residues previously shown to influence alcohol and anaesthetic action on these proteins. These results suggest a common structural basis for ethanol potentiation of an important class of targets for neurological actions of ethanol. Since the development of alcoholic fermentation technology millenia ago, ethanol has been one of the most widely used drugs in human civilization [1] . Today, the excessive use of ethanol imposes a considerable health and economic burden in many countries; among other things, it is the major global cause of disability in people 10–24 years of age [2] . Ethanol is unique among commonly used drugs in that its molecular sites and mechanisms of action are poorly defined, mainly owing to the weak binding energy of this small molecule and the lack of X-ray structures of alcohol bound to targets relevant for its intoxicating effects [3] . Similarities in the chemical and pharmacological profiles of alcohols and anaesthetics have led to the proposal that these agents may act via shared sites of action; however, the nature of these interactions remains unclear. Studies of neurological actions of alcohols and anaesthetics have focused on ligand-gated ion channels such as GABA(A), glycine and nicotinic acetylcholine receptors [3] . Several of these receptors are genetically linked to ethanol effects in animals [4] , [5] and humans [6] , and are modulated by alcohols and anaesthetics in vitro [7] , [8] , [9] , [10] , [11] . Receptors in this family are assembled from five identical or similar subunits arranged around a C5 symmetry axis perpendicular to the membrane; each subunit contains a large ligand-binding extracellular domain, a transmembrane domain comprised of four helices (M1–M4) from each subunit and a variable intracellular loop. These receptors carry neurotransmitter-binding sites within the extracellular domain, while the ion channel is located in the transmembrane domain. The coupling of agonist binding and channel opening involves critical regions between the extracellular and transmembrane domains, particularly extracellular loops 2 and 7 and the upper portion of the pore-lining M2 helices [12] . Mutagenesis and labelling studies have identified a few specific residues critical to alcohol and anaesthetic effects, primarily in the transmembrane domain [3] . However, in the absence of high-resolution structures of human ligand-gated ion channels, our understanding of the molecular effects of these agents remains limited compared with most other psychoactive drugs. A remarkable advance in our ability to study alcohol and anaesthetic modulation was the recent crystallization of ligand-gated ion channels from lower organisms that are closely related to mammalian targets of alcohol [13] , [14] , [15] , [16] . The proton-activated G. violaceus ligand-gated ion channel (GLIC) was crystallized in the presumed open state [17] , and has since been determined in an alternative ‘locally-closed’ conformation [18] , as well as in complex with various modulators [19] , [20] . In particular, GLIC exhibited inhibition by general anaesthetics [21] similar to nicotinic acetylcholine receptors [9] , and we determined its structure in complex with the anaesthetic agents propofol and desflurane [20] , providing insight into the structural basis for drug effects on some members of this family. More recently, we found that ethanol potentiates GLIC, though only at non-pharmacological concentrations [22] . In the GLIC structure, amino-acid positions implicated in alcohol modulation of human ligand-gated ion channels clustered around a set of inter- and intra-subunit transmembrane cavities [22] . Moreover, introduction of the mutation F238A in the pore-lining M2 helix (F14′A in prime notation, counting from the N terminus of M2) resulted in marked potentiation of function by pharmacologically relevant concentrations of ethanol [22] , similar to mammalian receptors. This ethanol-sensitized variant provides an opportunity to use structural methods to define the site(s) responsible for ethanol modulation of this and other ligand-gated ion channels. In this study, we determined crystal structures of the ethanol-sensitized GLIC variant in the absence and presence of ethanol and other modulators. These structures suggested a structural mechanism for stabilization of the open form of the channel by alcohols and anaesthetics. Mutations expected to alter modulator binding confirmed the importance of specific interactions revealed by the new structures. Multalignments and homology modelling indicated that a similar mode of binding is likely to exist in human ethanol-sensitive ligand-gated ion chanels, such as glycine and GABA(A) receptors. Crystal structure of a GLIC ethanol-sensitized variant Previous studies showed that the F14′A mutation in GLIC slightly reduces proton sensitivity (shifting EC 50 from pH 4.9 to pH 4.3) and dramatically enhances ethanol sensitivity, conferring potentiation by pharmacologically relevant (20 mM) concentrations of ethanol [22] . To investigate the structural basis for these changes, the structure of the ethanol-sensitized GLIC mutant F14′A was determined at 2.75 Å ( Supplementary Table S1 ) under crystallization conditions similar to those used in previous structures of wild-type GLIC ( Fig. 1a ) [14] . The mutant structure ( Fig. 1b ) was similar to that of the wild-type protein, with a root mean square deviation of 0.22 Å over the 1,555 Cα atoms. The principal structural difference was in the region of the 14′ residue, which in wild-type GLIC forms one end of a transmembrane cavity at the interface between channel subunits [20] ( Fig. 1a ). In the mutant structure, the absence of the phenyl ring at 14′ was associated with an expanded inter-subunit cavity, penetrating one to two registers deeper into the membrane-spanning region. The volume of the cavity was increased by 267 Å 3 . This cavity was relatively polar and likely to be hydrated; indeed, electron density for at least one water molecule was well resolved ( Fig. 1b ). The mutation also appeared to increase structural flexibility, as indicated by high B-factors throughout the structure (99.5 Å 2 ) ( Fig. 1b ) relative to the wild-type (69.6 Å 2 ) ( Fig. 1a ). Although many reasons could account for the B-factor deviations observed between the GLIC F14′A and wild-type structures, several observations suggest that these differences are specifically caused by the F14′A mutation: (1) Both proteins crystallize in the same space group, display identical unit cell dimensions and both structures were solved at similar resolutions. (2) The B-factor deviations were not homogeneously distributed over the protein; instead, they were concentrated in the transmembrane domain, especially in regions neighbouring the inter-subunit transmembrane cavity, including the extracellular portion of M2 and pre-M1. Deviations in B-factors were also observed in loops 2, 7 and F, connecting the extracellular to the transmembrane domains ( Supplementary Fig. S1 ). (3) The most affected region by the F14′A mutation lies about 35 Å from the closest crystal contact suggesting that the B-factor deviations are not owing to lattice disorders. (4) This structural destabilization of the presumed open conformation of GLIC might also explain the reduced proton sensitivity observed for this mutant [22] . 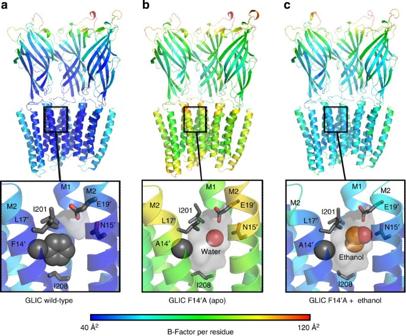Figure 1: X-ray structures of wild-type and ethanol-sensitized GLIC. (a) Wild-type GLIC (PDB ID 4HFI), coloured by residue B-factor according to scale at bottom. For clarity, proximal two subunits are hidden, revealing distal three subunits surrounding channel pore. Lower panel shows inter-subunit transmembrane cavity (light grey surface) formed by the extracellular portions of M1–M2 from one subunit and M2–M3 from the neighbouring subunit, and occluded on one end by the F14′ side chain (dark grey spheres). (b) Ethanol-sensitized GLIC variant (F14′A) (PDB ID 4HFB), depicted as ina. Lower panel shows expanded inter-subunit cavity containing resolved water (red sphere). (c) GLIC F14′A mutant co-crystallized with ethanol (PDB ID 4HFE), depicted as ina. Lower panel shows inter-subunit cavity containing ethanol (orange and red spheres). Figure 1: X-ray structures of wild-type and ethanol-sensitized GLIC. ( a ) Wild-type GLIC (PDB ID 4HFI), coloured by residue B-factor according to scale at bottom. For clarity, proximal two subunits are hidden, revealing distal three subunits surrounding channel pore. Lower panel shows inter-subunit transmembrane cavity (light grey surface) formed by the extracellular portions of M1–M2 from one subunit and M2–M3 from the neighbouring subunit, and occluded on one end by the F14′ side chain (dark grey spheres). ( b ) Ethanol-sensitized GLIC variant (F14′A) (PDB ID 4HFB), depicted as in a . Lower panel shows expanded inter-subunit cavity containing resolved water (red sphere). ( c ) GLIC F14′A mutant co-crystallized with ethanol (PDB ID 4HFE), depicted as in a . Lower panel shows inter-subunit cavity containing ethanol (orange and red spheres). Full size image Structures of the GLIC F14′A variant bound to alcohols We then grew crystals of the GLIC F14′A variant in the presence of ethanol, and determined the structure to 2.80 Å ( Supplementary Table S1 ). The ethanol-bound structure ( Fig. 1c ) was completely superimposable with the apo-form of F14′A, except for a strong Fo–Fc electron density peak in each of the expanded inter-subunit cavities (7.6±0.8 σ over all five monomers) ( Figs 2a and 3a and Supplementary Fig. S2a ). 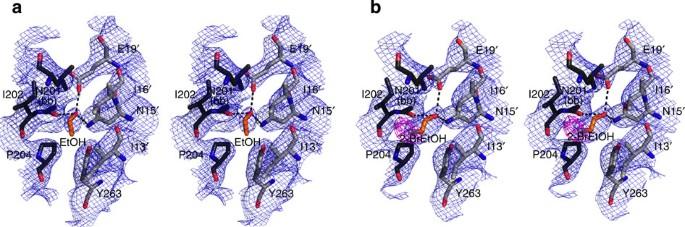Figure 2: Refinement of alcohol-binding site. (a) Stereo view of protein atoms neighbouring one ethanol molecule (orange) in the co-crystal structure with GLIC F14′A. Dotted lines indicate putative hydrogen bonds with the backbone carbonyl of N200 in the left-hand subunit (dark grey) and with N15′ and E19′ in the right-hand subunit (light grey). (b) Protein atoms neighbouring one molecule of 2-bromoethanol (orange) in the co-crystal structure with GLIC F14′A, displayed as ina. Sigma-A-averaged electron density surrounding ethanol and 2-bromoethanol are contoured at 1.0 σ (blue mesh) and bromine-anomalous map is contoured at 5.0 σ (magenta mesh). Figure 2: Refinement of alcohol-binding site. ( a ) Stereo view of protein atoms neighbouring one ethanol molecule (orange) in the co-crystal structure with GLIC F14′A. Dotted lines indicate putative hydrogen bonds with the backbone carbonyl of N200 in the left-hand subunit (dark grey) and with N15′ and E19′ in the right-hand subunit (light grey). ( b ) Protein atoms neighbouring one molecule of 2-bromoethanol (orange) in the co-crystal structure with GLIC F14′A, displayed as in a . Sigma-A-averaged electron density surrounding ethanol and 2-bromoethanol are contoured at 1.0 σ (blue mesh) and bromine-anomalous map is contoured at 5.0 σ (magenta mesh). 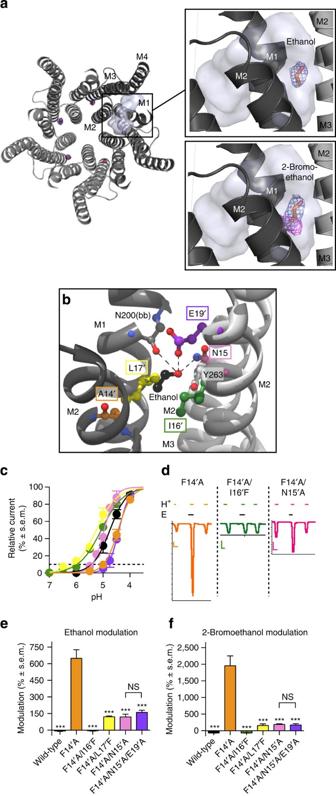Figure 3: Alcohol binding to ethanol-sensitized GLIC. (a) Left, extracellular view of full transmembrane domain showing the sigma-A-averaged 2Fo–Fc electron density map (blue) contoured at 1.0 σ surrounding the refined position of ethanol (orange). Top right, equivalent density relative to contiguous transmembrane cavities (white) associated with one subunit interface. Bottom right, same representation for GLIC F14′A co-crystallized with 2-bromoethanol. The 2Fo–Fc electron density (blue) is overlaid with bromine-specific anomalous map (magenta) contoured at 5.0 σ. All maps are pictured within 2 Å of the modelled ligands. (b) Inter-subunit interface of F14′A plus ethanol, showing M1–M2 (dark grey) and M2–M3 (light grey) from neighbouring subunits, backbone and side-chain atoms for interfacial 14′ residue, and all amino acids within 4 Å of ethanol. Dashes indicate three possible hydrogen bonds. Residue N200 neighbours ethanol via its backbone carbonyl, and only its backbone is shown. (c) Proton response curves for GLIC wild-type (black), F14′A (orange) and F14′A-containing mutants I16′F (green), L17′F (yellow), N15′A (pink) and N15′A/E19′A (purple). Dashes indicate EC10. (d) Sample traces showing EC10activations (H+) of GLIC F14′A, F14′A/I16′F and F14′A/N15′A in the absence and presence of 200 mM ethanol (E). Scale bars: 500 nA, 2 min. (e) Modulation by 200 mM ethanol of GLIC currents;n=5–16. (f) Modulation by 60 mM 2-bromoethanol, shown as inf;n=4–5. Infandg, bracket represents two-tailed unpairedt-test, not significant (NS); all other comparisons indicate analysis of variance, Dunnett’s test significance versus F14′A; ***P<0.001. Full size image Figure 3: Alcohol binding to ethanol-sensitized GLIC. ( a ) Left, extracellular view of full transmembrane domain showing the sigma-A-averaged 2Fo–Fc electron density map (blue) contoured at 1.0 σ surrounding the refined position of ethanol (orange). Top right, equivalent density relative to contiguous transmembrane cavities (white) associated with one subunit interface. Bottom right, same representation for GLIC F14′A co-crystallized with 2-bromoethanol. The 2Fo–Fc electron density (blue) is overlaid with bromine-specific anomalous map (magenta) contoured at 5.0 σ. All maps are pictured within 2 Å of the modelled ligands. ( b ) Inter-subunit interface of F14′A plus ethanol, showing M1–M2 (dark grey) and M2–M3 (light grey) from neighbouring subunits, backbone and side-chain atoms for interfacial 14′ residue, and all amino acids within 4 Å of ethanol. Dashes indicate three possible hydrogen bonds. Residue N200 neighbours ethanol via its backbone carbonyl, and only its backbone is shown. ( c ) Proton response curves for GLIC wild-type (black), F14′A (orange) and F14′A-containing mutants I16′F (green), L17′F (yellow), N15′A (pink) and N15′A/E19′A (purple). Dashes indicate EC 10 . ( d ) Sample traces showing EC 10 activations (H + ) of GLIC F14′A, F14′A/I16′F and F14′A/N15′A in the absence and presence of 200 mM ethanol (E). Scale bars: 500 nA, 2 min. ( e ) Modulation by 200 mM ethanol of GLIC currents; n =5–16. ( f ) Modulation by 60 mM 2-bromoethanol, shown as in f ; n =4–5. In f and g , bracket represents two-tailed unpaired t- test, not significant (NS); all other comparisons indicate analysis of variance, Dunnett’s test significance versus F14′A; *** P <0.001. Full size image Identifying the position and orientation of ethanol by X-ray crystallography is particularly challenging owing to its small size, lack of distinguishing structural features and weak binding energy. Therefore, in order to confirm the presence and structure of ethanol in the electron density, we repeated the experiment using 2-bromoethanol, an analogue of ethanol containing a bromine atom that produces a specific anomalous signal that can be observed by crystallography using X-rays with tunable wavelengths. A 3.05 Å structure ( Supplementary Table S1 ) of GLIC F14′A co-crystallized with 2-bromoethanol contained the same peak in the Fo–Fc electron density, as well as a strong bromine anomalous signal (5.4±0.5 σ over all five monomers) overlapping the most buried portion of the peak ( Figs 2b and 3a , Supplementary Fig. S2b ). We therefore assigned the inter-subunit density to one ethanol molecule per subunit, each oriented with its aliphatic chain buried in the cavity, and its hydroxyl group facing towards the transmembrane/extracellular domain interface ( Fig. 3b ). The inter-subunit ethanol-binding cavity was distinct from the intra-subunit cavity previously shown to bind inhibitory anaesthetics [20] in wild-type GLIC. In addition, the presence of a weak intra-subunit bromine anomalous signal in the co-crystal structure with 2-bromoethanol supported the possibility that alcohols may also bind there, but with too low occupancy or too high mobility to allow for confident model building ( Supplementary Figs S2a, S2b ). Co-crystallization with ethanol appeared to stabilize the F14′A structure, resulting in decreased overall B-factors (85.5 Å 2 ) with a distribution that resembled wild-type GLIC ( Fig. 1c and Supplementary Fig. S1 ). Given that GLIC was crystallized under activating conditions (pH 4.0), has a pore wide enough to conduct ions [17] , and corresponds to other recent open structures of ligand-gated ion channels [16] , the decrease in B-factors upon ethanol binding would be consistent with a macroscopic role for the drug in stabilizing the open state of the channel. Nevertheless, other experiments will be necessary to formally demonstrate that point. The structural data suggest that ethanol potentiates the GLIC F14′A mutant by binding to the expanded inter-subunit cavity. In order to test this hypothesis, we performed site-directed mutagenesis of residues bordering the ethanol-binding pocket that was observed by crystallography. Mapping the ethanol-binding site by site-directed mutagenesis Ethanol binding was mediated by hydrophobic and hydrophilic interactions. The closest hydrophobic contacts of the aliphatic chain were with residue I16′ in the M2 helix of one subunit and L17′ in M2 of the neighbouring subunit ( Fig. 3b ). Substituting phenylalanine at either of these positions compensated for reduced proton sensitivity of the F14′A variant ( Fig. 3c ) and reduced the effect of F14′A on modulation by both ethanol ( Fig. 3d ) and 2-bromoethanol ( Fig. 3f ): L17′F reduced potentiation more than fivefold, while I16′F blocked potentiation entirely, resulting in a channel similar to wild-type GLIC. Our co-crystal structure also revealed three possible hydrogen bonds with the ethanol hydroxyl group ( Fig. 3b ). Owing to a conserved proline in the n +4 position [23] , the carbonyl oxygen of M1 residue N200 is kinked towards the inter-subunit cavity, and is in a position to accept a hydrogen bond from ethanol in the co-crystal structure or from water in the apo-structures. The ethanol hydroxyl group also borders the M2 residue N15′, which could donate or accept a hydrogen bond, and which aligns with the most critical residue for alcohol potentiation of GABA(A) and glycine receptors [24] . Disrupting hydrogen bonding by substituting alanine at N15′ in the context of F14′A compensated for reduced proton sensitivity ( Fig. 3c ) and decreased potentiation by ethanol ( Fig. 3d ) and 2-bromoethanol ( Fig. 3f ), consistent with a role for this interaction in stabilizing alcohol binding and modulation. We also tested a potential hydrogen bond with residue E19′ at the extracellular end of the inter-subunit cavity. As the double mutant F14′A/E19′A was non-functional, we characterized the triple mutant F14′A/N15′A/E19′A, in which disruption of the E19′ interaction did not further decrease ethanol ( Fig. 3e ) nor 2-bromoethanol ( Fig. 3f ) potentiation, compared with F14′A/N15′A. Thus, the N15′ interaction appeared to be particularly critical for alcohol binding. Polar interactions at this site may be important, given that a water molecule was resolved in the equivalent region of the GLIC F14′A apo-structure ( Fig. 1b ). Overlapping binding of general anaesthetics To better understand the mechanism for allosteric modulation by alcohols and related anaesthetic agents, we determined additional crystal structures ( Supplementary Table S1 ) of the volatile anaesthetic bromoform bound to both wild-type GLIC ( Fig. 4a ) and the ethanol-sensitized variant ( Fig. 4b ). Bromoform is a structural analogue of chloroform, in which the chlorine atoms are substituted by bromine, thereby producing a specific anomalous signal that allows the unambiguous localization of the molecule in the electron density. Like other volatile anaesthetics [21] , bromoform inhibited wild-type GLIC ( Fig. 4c ); the current work confirms and extends, by making use of a higher resolution and the bromine-specific anomalous signal ( Fig. 4a and Supplementary Fig. S2d ), the earlier observation of propofol and desflurane [20] binding into the intra-subunit cavity. Indeed, this higher-resolution structure reveals that bromoform occupy alternatively three poses in the intra-subunit cavity, including two poses close to the original ones. The first two poses of bromoform were modelled and refined as alternative conformations of the same bromoform molecule. The third pose has a markedly lower occupation and anomalous signal. 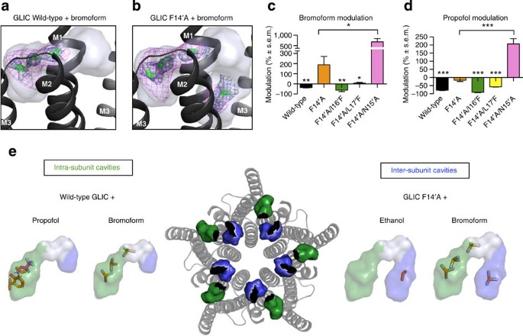Figure 4: Bromoform binding to wild-type and ethanol-sensitized GLIC. Bromine-specific anomalous map contoured at 5.0 σ (magenta) and sigma-A-averaged 2Fo–Fc electron density map (blue) assigned to bromoform (green) relative to the contiguous intra- and inter-subunit transmembrane cavities (white) associated with one subunit interface of wild-type GLIC (a) and the ethanol-sensitized GLIC variant (F14′A) (b). The anomalous and 2Fo–Fc maps are, respectively, pictured within 4 and 2 Å of the modelled ligands. (c) Modulation by 1 mM bromoform of GLIC wild-type (black), F14′A (orange), and F14′A-containing mutants I16′F (green), L17′F (yellow) and N15′A (pink); left axis broken for clarity;n=5–8. (d) Modulation by 100 μM propofol of GLIC variants as inc;n=5–11. Incandd, bracket represents significant difference between GLIC F14′A and F14′A/N15′A measured by two-tailed unpairedt-test; all other comparisons indicate analysis of variance, Dunnett’s test significance versus F14′A; *P<0.05, **P<0.01, ***P<0.001. (e) The intra- (green) and inter-subunit (blue) cavities associated with a single-subunit interface from the indicated co-crystal structure. Inset structures represent wild-type GLIC co-crystallized with inhibitory anaesthetics, which overlap the previously described propofol- (orange) and desflurane (pink)-binding sites20. Inter-subunit sites (blue) associated with receptor potentiation. Insets represent GLIC F14′A structures crystallized with potentiating agents. Figure 4: Bromoform binding to wild-type and ethanol-sensitized GLIC. Bromine-specific anomalous map contoured at 5.0 σ (magenta) and sigma-A-averaged 2Fo–Fc electron density map (blue) assigned to bromoform (green) relative to the contiguous intra- and inter-subunit transmembrane cavities (white) associated with one subunit interface of wild-type GLIC ( a ) and the ethanol-sensitized GLIC variant (F14′A) ( b ). The anomalous and 2Fo–Fc maps are, respectively, pictured within 4 and 2 Å of the modelled ligands. ( c ) Modulation by 1 mM bromoform of GLIC wild-type (black), F14′A (orange), and F14′A-containing mutants I16′F (green), L17′F (yellow) and N15′A (pink); left axis broken for clarity; n =5–8. ( d ) Modulation by 100 μM propofol of GLIC variants as in c ; n =5–11. In c and d , bracket represents significant difference between GLIC F14′A and F14′A/N15′A measured by two-tailed unpaired t- test; all other comparisons indicate analysis of variance, Dunnett’s test significance versus F14′A; * P <0.05, ** P <0.01, *** P <0.001. ( e ) The intra- (green) and inter-subunit (blue) cavities associated with a single-subunit interface from the indicated co-crystal structure. Inset structures represent wild-type GLIC co-crystallized with inhibitory anaesthetics, which overlap the previously described propofol- (orange) and desflurane (pink)-binding sites [20] . Inter-subunit sites (blue) associated with receptor potentiation. Insets represent GLIC F14′A structures crystallized with potentiating agents. Full size image The F14′A mutation converted bromoform into a potentiator, as with long-chain alcohols [22] ( Fig. 4c ). In this case, bromoform was found to bind not only to the previously known intra-subunit cavity but also to the inter-subunit cavity described here for ethanol ( Fig. 4b , Supplementary Fig. S2c ). In addition, the crystal structure reveals that bromoform adopts different ‘binding-modes’ in the intra- and inter-subunit cavities. In the intra-subunit cavity, bromoform displays a substantial mobility and occupies alternatively different poses. This is reminiscent of previously published functional and structural data that suggested a significant mobility of propofol and desflurane in this cavity [20] . In the inter-subunit cavity, the volume and shape of the cavity imposes one pose for bromoform, which was refined with a full occupancy. Interestingly, binding of bromoform to the F14′A ethanol-sensitized mutant produced the same macroscopic-stabilizing effect on the B-factor distribution that was observed for the ethanol-bound structure (data not shown). As for ethanol, these results suggest that potentiation by bromoform of the GLIC ethanol-sensitized mutant occurs through binding in the inter-subunit cavity of the open channel. Phenylalanine substitutions in the inter-subunit site blocked potentiation of the GLIC variant by bromoform ( Fig. 4c ), indicating that the anaesthetic and alcohols occupied overlapping potentiating sites. A similar pattern was observed for propofol inhibition, which was blocked by the F14′A mutation and restored by phenylalanine substitutions in the inter-subunit site ( Fig. 4d ). Interestingly, while the hydrophilic N15′ interaction was critical for ethanol potentiation, substituting alanine at this residue further enhanced potentiation by bromoform ( Fig. 4c ) and propofol ( Fig. 4d ). This pattern is consistent with the hydrophobic nature of anaesthetics, including bromoform and propofol, relative to ethanol, such that they may depend more heavily on van der Waals interactions within the protein-binding site. These observations support an overlapping but chemically distinct mechanism of allostery by anaesthetics compared with alcohol. Ethanol has been co-crystallized as a solvent or cofactor in several other published protein structures, including mammalian alcohol dehydrogenase as early as 1994 (ref. 25 ). Among proteins implicated in neurological effects of ethanol, structural information has been limited to the Drosophila protein LUSH [26] (not observed in humans), although a larger alcohol was co-crystallized with the isolated cytoplasmic domain of an inwardly rectifying potassium channel (IRK1) [27] . In the apo form, LUSH displays conformational flexibility, but is rigidified upon binding of alcohols via a central hydrophobic pocket of the protein, as demonstrated by peak narrowing in NMR spectra [26] . Consistent with the types of molecular interactions observed in LUSH [26] and IRK1 (ref. 27 ), ethanol interacted with the GLIC variant via multiple hydrophobic contacts and at least one hydrogen bond. Although other experiments will be necessary to further document that point, the crystal structure suggests that ethanol binding to the GLIC ethanol-sensitive mutant stabilizes the open conformation of the channel as indicated by a marked decrease of B-factors within the region of the ethanol-binding pocket. Our structural data showed that potentiation by alcohol and anaesthetics occurrs upon binding into an inter-subunit cavity in GLIC F14′A, directly stabilizing the open state of the channel. This observation is supported by site-directed mutagenesis experiments based on the GLIC F14′A structures, revealing that phenylalanine substitutions at either the 16′ or 17′ positions (both proximal to the ethyl carbons of ethanol) blocked the inter-subunit cavity and disrupted potentiating interactions with ethanol and general anaesthetics. Moreover, both substitutions enhanced proton sensitivity, reflecting that channel opening is facilitated by decreased volume and/or increased hydrophobic contacts in the inter-subunit cavity [18] . Substitution of alanine at N15′ could also increase hydrophobic interactions at the subunit interface, resulting in a similarly decreased EC 50 for proton. Notably, these results suggest that the mechanism of open state stabilization via mutations is at least partially shared with that of alcohol potentiation. Previous cysteine labelling at positions 17′–19′ appeared to mimic ethanol potentiation [22] further supporting a model in which occupation of the inter-subunit pocket promotes channel opening in GLIC (ref. 18 ). This study also confirmed that alcohols and anaesthetics share sites of action on ligand-gated ion channels. Indeed, resolution of the volatile anaesthetic bromoform in the inter-subunit cavity of GLIC F14′A—overlapping the position of ethanol and relying to a similar extent on the hydrophobic 16′ and 17′ residues—indicated that the enhanced inter-subunit ethanol-binding site also facilitated an inter-subunit-binding mode for anaesthetics. Notably, bromoform has no hydroxyl moiety, and was therefore incapable of hydrogen bonding with the 15′ residue; generally, hydrophobic interactions are likely to have a bigger role in anaesthetic binding versus alcohols, which may rely more on hydrogen bonding. This distinction may explain the opposite effects of the N15′A mutation on alcohol versus anaesthetic modulation: loss of the N15′ hydrogen bond correlated with reduced alcohol potentiation, whereas the nonpolar residue substitution here increased anaesthetic potentiation. Our data suggest that binding of anaesthetics and alcohols may be structurally overlapping, yet chemically distinct. Combined structural and mutational data strongly support that the inter-subunit cavity mediates the potentiating effects of ethanol and anaesthetics. Our previous structural studies suggest that the intra-subunit cavity is important for inhibition of channel function [20] . However, binding of anaesthetics to the intra-subunit cavity was observed in the structure of the open form of the channel, whereas anaesthetics are expected to stabilize a closed form. One possibility is that this intra-subunit cavity is remodelled upon the transition towards a closed form of the channel so that the anaesthetics can bind more strongly to the closed form than to the open form. In support of this idea, recent results from a photoreactive activable propofol analogue suggest that propofol binds to a similar inhibitory intra-subunit cavity preferentially in a desensitized closed form of the nicotinic acetylcholine receptor [28] . Definitive characterization of channel inhibition mechanisms will likely require determination of high-resolution co-crystal structures of the closed channel bounds to anaesthetics. The novel potentiating site identified in the GLIC variant structure occupies a pivotal location for gating at the interface of TMD subunits and ECD–TMD domains. Moreover, this pocket contacts the extracellular half of the M2 helices; this region was shown to have a key role in gating in the recently determined non-conductive state of GLIC, which displayed a conserved alternative conformation in M2 and an expanded inter-subunit cavity [18] . This potentiating site also overlaps the allosteric agonist ivermectin in recent structures of the Caenorhabditis elegans glutamate-gated chloride channel [16] . However, ivermectin binding produces a local displacement of the M1 and M3 transmembrane helices within the three-dimensional structure, while in our case ethanol binding preserves the conformation intact but apparently provides energetic stabilization. These data thus suggest an overlapping inter-subunit location, but different mechanisms for stabilizing the open state of ligand-gated ion channels by the small (46 Da) ethanol and the relatively large (875 Da) ivermectin molecules. The GLIC F14′A variant is a structural and functional homologue of known neurological targets of alcohol and anaesthetics, particularly GABA(A) and glycine receptors, which mediate fast inhibitory neurotransmission in the brain and spinal cord. Ethanol enhances the depressant effects of both GABA (ref. 29 ) and glycine [30] in mice, and genetic studies support the involvement of GABA(A) and glycine receptors in behavioural effects of ethanol in animals [4] . In addition, the α2 and γ1 subtypes of GABA(A) receptors are associated with genetic risk for alcohol dependence in humans [6] . In heterologous expression systems, some members of these receptor families are potentiated by 30–100 mM ethanol, concentrations that produce moderate to severe intoxication in humans [3] . A similar range of approaches identified GABA(A) and glycine receptors as substrates for general anaesthetics [11] . In most cases, anaesthetics resemble ethanol in potentiating GABA(A) and glycine receptor function, including volatile and injected anaesthetics and a wide range of n -alcohols [7] , [8] , [10] . Molecular studies have proposed extracellular [31] , [32] , intracellular [33] and transmembrane [24] sites of action for alcohols and anaesthetics in GABA(A) and glycine receptors. Our work supports the proposed transmembrane mechanism, as we observed ethanol binding exclusively in this region; this is consistent with previous studies of a GLIC/glycine receptor chimera that demonstrated that the transmembrane domain is sufficient to confer alcohol and anaesthetic modulation properties [34] . Superposition of the ethanol-binding pocket identified in our study onto a homology model of the human α1 glycine receptor [35] revealed a large inter-subunit cavity capable of accommodating ethanol ( Fig. 5b ). Striking similarities are observed between both receptors, including conservation of an unbonded backbone carbonyl in M1 and of polar residues at both the 15′ and 19′ putative hydrogen-bonding side chains ( Fig. 5a ). Furthermore, hydrophobic contacts limiting the size of the inter-subunit cavity in the GLIC variant (I16′ and L17′) were absent in the glycine receptor model (S16′ and G17′) ( Fig. 5b ), suggesting a structural basis for sensitivity of glycine receptors to potentiation by larger alcohols [7] . Indeed, sequence alignments indicated that all four residues implicated in ethanol action in this study—positions 14′–17′—are smaller and, in several cases, more hydrophilic in GABA(A) and glycine receptors than in wild-type GLIC, and could account for the greater ethanol sensitivity and higher cutoff for n -alcohol potentiation exhibited by these human receptors [7] , [8] relative to GLIC [22] . Recent molecular dynamic simulations also illustrated spontaneous interactions of ethanol with the inter-subunit cavity of a glycine receptor homology model [36] , consistent with our more recent results with GLIC F14′A and supporting the generalizability of this model system to human inhibitory receptors. 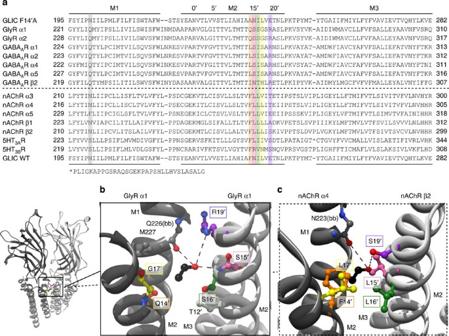Figure 5: Alignment of GLIC F14′A with human alcohol targets. (a) Sequence alignment of GLIC M1–M3 helices with human ethanol-sensitive ligand-gated ion channels. M2 residues 14′, 15′, 16′, 17′ and 19′ coloured as inFig. 2b; carbonyl of M1 residue equivalent to GLIC N200 (grey) is available to interact with solvent owing to a conserved proline in then+4 position. Receptors above dashes exhibit high ethanol sensitivity and/or longer cutoffs forn-alcohol potentiation; receptors below exhibit limited ethanol sensitivity and inhibition by long-chainn-alcohols. (b) View as inFig. 2bof a human α1 glycine receptor (GlyRα1) homology model based on GLIC (PDB ID 3EAM) as previously described35, with ethanol as in the F14′A co-crystal structure. Ribbons represent M1–M2 (dark grey) and M2–M3 (light grey) from neighbouring subunits. Amino acids within 4 Å of superimposed ethanol molecule (Q226, M227, T12′, Q14′, S15′, S16′ and R19′), as well as G17′, are shown as balls-and-sticks. Only backbone atoms of Q226 (equivalent to GLIC N200) are shown. Backbone and side-chain atoms for residues S15′ and G17′ are shown for clarity. (c) View as inFig. 2aof a model of the human α4β2 nicotinic acetylcholine receptor, generated by superimposing human α4 (PDB ID 2LLY) and β2 (PDB ID 2LM2) nicotinic acetylcholine receptor subunits on the GLIC F14′A ethanol co-crystal structure backbone. Amino acids within 4 Å of the superimposed ethanol molecule (F14′, L15′and L17′), as well as L16′, S19′, and backbone atoms of residue N223 (equivalent to GLIC N200), are shown as balls-and-sticks. Figure 5: Alignment of GLIC F14′A with human alcohol targets. ( a ) Sequence alignment of GLIC M1–M3 helices with human ethanol-sensitive ligand-gated ion channels. M2 residues 14′, 15′, 16′, 17′ and 19′ coloured as in Fig. 2b ; carbonyl of M1 residue equivalent to GLIC N200 (grey) is available to interact with solvent owing to a conserved proline in the n +4 position. Receptors above dashes exhibit high ethanol sensitivity and/or longer cutoffs for n -alcohol potentiation; receptors below exhibit limited ethanol sensitivity and inhibition by long-chain n -alcohols. ( b ) View as in Fig. 2b of a human α1 glycine receptor (GlyRα1) homology model based on GLIC (PDB ID 3EAM) as previously described [35] , with ethanol as in the F14′A co-crystal structure. Ribbons represent M1–M2 (dark grey) and M2–M3 (light grey) from neighbouring subunits. Amino acids within 4 Å of superimposed ethanol molecule (Q226, M227, T12′, Q14′, S15′, S16′ and R19′), as well as G17′, are shown as balls-and-sticks. Only backbone atoms of Q226 (equivalent to GLIC N200) are shown. Backbone and side-chain atoms for residues S15′ and G17′ are shown for clarity. ( c ) View as in Fig. 2a of a model of the human α4β2 nicotinic acetylcholine receptor, generated by superimposing human α4 (PDB ID 2LLY) and β2 (PDB ID 2LM2) nicotinic acetylcholine receptor subunits on the GLIC F14′A ethanol co-crystal structure backbone. Amino acids within 4 Å of the superimposed ethanol molecule (F14′, L15′and L17′), as well as L16′, S19′, and backbone atoms of residue N223 (equivalent to GLIC N200), are shown as balls-and-sticks. Full size image Our results with GLIC F14′A are consistent with specific amino-acid interactions previously shown to control allosteric modulation of GABA(A) and glycine receptors. Past studies noted that bulkier substitutions at the 14′ position of β2 GABA(A) receptors [37] and α1 glycine receptors [35] reduced anaesthetic and ethanol sensitivity, respectively. Photo-labelling experiments localized an etomidate photo-reactive analogue-binding site in a cavity located at the transmembrane interface between subunits [38] . Moreover, the 15′ residues in both receptor families were found to be critical for alcohol and anaesthetic modulation [24] , [39] , echoing our structural and functional evidence for a critical hydrogen bond between ethanol and the 15′ residue in GLIC F14′A. In contrast to the GLIC F14′A variant, wild-type GLIC functional properties resemble several aspects of nicotinic acetylcholine receptors, which have an excitatory role in neurotransmission and modulation. Evidence for alcohol action at nicotinic receptors includes cross-tolerance and twin studies linking it to nicotine use, as well as genetic changes in the neuronal (α4β2) nicotinic receptor that influence behavioural effects of ethanol [5] . At the physiological level, ethanol potentiates α4β2 nicotinic currents in cortical and heterologous cell systems; however, these receptors were inhibited rather than potentiated by long-chain n -alcohols and general anaesthetics [9] —a pattern similar to wild-type GLIC, with a slightly higher n -alcohol cutoff for potentiation [22] . Superimposing α4β2 nicotinic acetylcholine receptor subunits from recent NMR structures [40] on the GLIC F14′A backbone revealed a cluster of large hydrophobic residues surrounding the inter-subunit cavity ( Fig. 5c ). In particular, the F14′ residue from wild-type GLIC is conserved in nicotinic receptor subunits, and the N15′ hydrogen bond partner is replaced by L15′ ( Fig. 5c ). Previous studies showed that the 15′ residue does not mediate ethanol potentiation in nicotinic receptors; instead, the 16′ and 17′ residues influence alcohol inhibition and potentiation, respectively [41] . Thus, amino-acid variations may produce a smaller, more hydrophobic inter-subunit cavity in nicotinic versus GABA(A) and glycine receptors, and could account for their lower cutoff for n -alcohol potentiation [9] . In conclusion, this work provides novel structural and functional insights into the potentiation by alcohols and anaesthetics of a ligand-gated ion channel. Examination of sequence data in a structural framework suggest that there is a common mode of action for human receptors, thus opening the way to the rational design of novel allosteric modulators of members of this family of cys-loop receptors. Reagents Chemicals were purchased from Sigma-Aldrich. The bromoform test condition was chosen as the concentration required to inhibit wild-type GLIC currents by ~50%, and was equal to the anaesthetic dose (minimum alveolar concentration required to eliminate response to a noxious stimulus in 50% of subjects, derived as previously described [42] ) of its analogue, chloroform, adjusted to deliver the reported concentration calibrated by gas chromatography [43] . At the time of application, the adjusted bromoform volume was added via positive displacement pipette to the appropriate Ringer’s buffer in a scintillation vial with minimal head space, immediately sealed with parafilm and aluminium foil, and sonicated for ≥2 min. The solution was applied by piercing the seal with the perfusion input needle, minimizing exposure of the solution surface to atmosphere. Propofol was prepared as 100 mM stock solution in dimethyl sulphoxide and used at 1000 × dilution after ≥2-min sonication. All modulators were diluted into fresh Ringer’s buffer at the time of electrophysiology. Protein expression and purification For crystallization, GLIC wild-type and F14′A variant were produced and purified as previously described [18] , [22] . Fractions corresponding to the predicted size of the pentameric protein were pooled and concentrated for crystallization. The GLIC F14′A variant behaved like the wild-type protein throughout the purification. For electrophysiology, expression plasmids containing wild-type GLIC in the pMT3 vector were prepared as previously described [44] . Mutagenesis was carried out using the QuikChange II site-directed mutagenesis kit (Agilent) using commercially made mutagenic primers (IDT). Mutant complementary DNA was confirmed by automated fluorescent DNA sequencing. Protein crystallization GLIC wild-type and F14′A variant were crystallized using vapour diffusion in hanging drops at 20 °C. The concentrated (8–12 mg ml −1 ) protein was mixed in a 1:1 ratio with reservoir solution containing typically 12–16% PEG 4000, 400 mM NaSCN and 0.1 M NaAc pH 4.0. Crystals appeared overnight in a parallepiped-like shape and grew for 1 week before reaching their final dimensions (typically 200 μm × 200 μm × 100 μm). Co-crystal structures were obtained by growing crystals in 200 mM ethanol, 200 mM 2-bromoethanol or 2% w/v bromoform. All crystals were cryoprotected using 20% glycerol and flash-frozen in liquid nitrogen. Crystallographic data collection All data sets were collected on beamline Proxima-I of the Soleil Synchrotron. For the crystals grown in complex with 2-bromoethanol and bromoform, data sets were collected at the peak wavelength of bromine (0.9191 Å), using the inversed-beam strategy in order to optimize the anomalous signal. For each structure presented in this work, ligand-binding sites deduced from a minimum of three different crystals diffracting at similar resolution were identical, supporting the reproducibility of these results. Reflections were integrated using XDS [45] and further analysed using the CCP4 programs [46] . Mutant and co-crystals were isomorphous to wild-type in the C2 space group with one pentamer in the asymmetric unit. Data collection statistics are summarized in Supplementary Table S1 . Phasing and refinement The structure of GLIC (PDB ID 3HFI) served as a starting model that was improved by alternate cycles of manual building in COOT [47] and refinement using REFMAC [48] and BUSTER (Global Phasing Ltd.). Ligand-binding sites were unambiguously identified in the electron density using the bromine-specific anomalous signal produced by the brominated ligands ( Supplementary Fig. S2 ). All ligands were refined with a full occupancy except for the three alternative binding sites of bromoform in the intra-subunit cavity, which were built with a partial occupancy that was refined in BUSTER. B-factors of 2-bromo-ethanol and bromoform deviated significantly from the protein B-factors ( Supplementary Table S1 ). Such B-factor deviation was already observed in other anaesthetic-bound structures of GLIC [20] and accounted for by a substantial mobility of these molecules that interact predominantly with the protein through hydrophobic contacts. In addition, high B-factors could also be owing to a partial loss of occupancy that occurred during data collection following bromine–carbon bond cleavage owing to irradiation damage, event though the effect of radiation damage was limited in our experiments by using an inversed-beam strategy for data collection. Non-crystallographic symmetry restraints and one translation libration screw parameter per protein chain were used throughout the refinement. Among the refined protein residues, 97.9–98.6% were in the most favoured regions of the Ramachandran plot, with 0% outliers. MolProbity scores [49] for the refined models all ranged within the 100th percentiles of structures refined at comparable resolutions. Details of the refinement statistics are provided in Supplementary Table S1 . We noted that 72 atoms corresponding to six detergent molecules resolved in the pore of wild-type GLIC were not observed in the F14′A mutant structure, possibly owing to the increased protein motion in this region indicated by increased B-factors. Pore density attributed to detergent molecules was restored in co-crystal structures with ethanol, 2-bromoethanol and bromoform, consistent with overall stabilization of the mutant channel pore region in the presence of allosteric modulators. Oocyte preparation Extraction of ovarian tissue from Xenopus laevis frogs was in accordance with the National Institutes of Health guide for the care and use of laboratory animals. Tissue was placed in Modified Barth’s Solution containing 88 mM NaCl, 10 mM HEPES, 2.4 mM NaHCO 3 , 1 mM KCl, 0.91 mM CaCl 2 , 0.82 mM MgSO 4 and 0.33 mM Ca(NO 3 ) 2 , adjusted to pH 7.5. After manual isolation with forceps, oocytes were treated with collagenase type 1A solution containing 0.5 mg ml −1 collagenase, 83 mM NaCl, 5 mM HEPES, 2 mM KCl and 1 mM MgCl 2 , adjusted to pH 7.5 for 10 min. Oocyte nuclei were injected via the animal pole with GLIC wild-type or mutant cDNA using a Nanoject II microdispenser (Drummond Scientific). Injected oocytes were singly stored at 13 °C in Modified Barth’s Solution supplemented with 220 mg l −1 sodium pyruvate, 90 mg l −1 theophylline, 50 mg l −1 gentamicin, 10 mg l −1 streptomycin and 10,000 U l −1 penicillin for 2–17 days. Electrophysiology Oocytes were placed in chambers (~100 μl volume) and perfused (2.0 ml min −1 ) with Ringer’s buffer (123 mM NaCl, 10 mM HEPES, 2 mM KCl, 2 mM MgSO 4 and 2 mM CaCl 2 ) using a peristaltic pump through 18-gauge Teflon and Viton tubing (Cole-Parmer). Oocytes were impaled with two glass electrodes filled with 3 M KCl and clamped at −70 mV using an OC-725C oocyte clamp (Warner Instruments). Currents were digitized and continuously plotted using the PowerLab 4/30 data acquisition system (AD Instruments). To activate GLIC currents, low-pH Ringer’s buffer was applied in which HEPES was replaced either with 10 mM citrate (pH 3.5–6.0) or 10 mM MOPS (pH 6.5–7.0). Proton activation curves ( Fig. 2c ) represent nonlinear regression fits to the equation R = R max /(1+10 ^ {[log(EC 50 − P )] n H }), where R is the peak channel response, R max is the maximal response, P is the concentration of protons, EC 50 is the concentration producing 50% maximal response and n H is the Hill coefficient. Data for each receptor were normalized to its fitted maximal response. To correct for effects on channel gating, we calculated the ~10% activation level of each mutant and used the corresponding pH to measure modulation. To quantify modulation, oocytes were treated for 1 min with low-pH Ringer’s buffer; after 5-min washout, the alcohol or anaesthetic solution was applied in neutral Ringer’s buffer for 1 min, then in low-pH buffer for 1 min; after another 5-min washout, low-pH buffer was again applied alone. Percentage modulation was calculated as [( R A − R 0 , R 1 ) / R 0 , R 1 ] × 100, where R A represents the channel response in the presence of modulator and R 0 , R 1 represents the mean of the pre- and post-modulator responses. Results were analysed with one-way analysis of variance and Dunnet’s post hoc test or by two-tailed unpaired t- test as appropriate, with significant effects set at P <0.05. Molecular modelling and visualization Figures were made using PyMol (Schrödinger) or UCSF Chimera [50] . Surface and size of the cavities were calculated using the Hollow script [51] . A homology model of the α1 glycine receptor ( Fig. 3b ) was built as previously described [35] by threading, refinement and molecular dynamics on the backbone of wild-type GLIC (PDB ID 3EAM) [14] using the Modeler module of Discovery Studio 2.5 (Accelrys), and aligned to the GLIC F14′A+ethanol co-crystal structure using the ‘match’ command in Chimera to perform least-squares fitting of all backbone atoms. The α4β2 nicotinic acetylcholine receptor ( Fig. 3c ) was roughly modelled using the ‘match’ command in Chimera to perform least-squares fitting of backbone atoms in M1(222–236) and M2(1′–19′) of a representative structure of the α4 nicotinic acetylcholine receptor subunit (PDB ID 2LLY) [40] to M1(199–213) and M2(1′–19′) in the B chain of the GLIC F14′A structure determined in the presence of ethanol (PDB ID 4HFE), and of M2(1′–19′) and M3(275–295) of a representative structure of the β2 subunit (PDB ID 2LM2) [40] to M2(1′–19′) and M3(258–278) in the C chain of GLIC F14′A+ethanol. As the determination of the nicotinic acetylcholine receptor subunit structures as monomers leaves substantial uncertainty about the packing of adjacent subunits, we limited our interpretation of this model to comparison of properties of directly aligned residues. How to cite this article: Sauguet, L. et al . Structural basis for potentiation by alcohols and anaesthetics in a ligand-gated ion channel. Nat. Commun. 4:1697 doi: 10.1038/ncomms2682 (2013).